Virus-like glycodendrinanoparticles displaying quasi-equivalent nested polyvalency upon glycoprotein platforms potently block viral infection Ligand polyvalency is a powerful modulator of protein–receptor interactions. Host–pathogen infection interactions are often mediated by glycan ligand–protein interactions, yet its interrogation with very high copy number ligands has been limited to heterogenous systems. Here we report that through the use of nested layers of multivalency we are able to assemble the most highly valent glycodendrimeric constructs yet seen (bearing up to 1,620 glycans). These constructs are pure and well-defined single entities that at diameters of up to 32 nm are capable of mimicking pathogens both in size and in their highly glycosylated surfaces. Through this mimicry these glyco-dendri-protein-nano-particles are capable of blocking (at picomolar concentrations) a model of the infection of T-lymphocytes and human dendritic cells by Ebola virus. The high associated polyvalency effects (β>10 6 , β/N ~10 2 –10 3 ) displayed on an unprecedented surface area by precise clusters suggest a general strategy for modulation of such interactions. The initial stages of an infectious process are crucial for subsequent immune response and elimination of pathogens [1] . The innate immune system comprises mechanisms and specialized cells responsible for first contact with external biological agents [2] . Detection of invaders via pathogen recognition receptors and subsequent activation of antimicrobial defences triggers specific antigen responses [3] . DC-SIGN (dendritic cell-specific intercellular adhesion molecule-3-grabbing nonintegrin) receptor is one of the most important pathogen recognition receptor. It is expressed mainly on the surface of dendritic cells (DCs), and some subtypes of macrophages [4] . DC-SIGN recognizes in a multivalent manner mannose and fucose containing glycoproteins [5] , such as ICAM-3 (intercellular adhesion molecule 3) present in T cells, and envelope glycoproteins found on pathogens [6] . By using DC-SIGN as an entry point some viruses are capable of escaping from the processing and degradation events carried out by the immune defence machinery at antigen-presenting cells [7] . Therefore, the inhibition of pathogen entry through the blockade of this receptor at early stages of infection is one strategy for new antiviral agents. Several studies have been directed towards the preparation of synthetic carbohydrate systems able to block or stimulate DC-SIGN [8] , [9] , [10] , [11] , [12] , [13] , [14] , [15] , [16] , [17] , [18] , [19] , [20] , [21] . Despite their elegant design, one of the problems that these artificial systems face is achieving adequate size and multivalency to sufficiently mimic natural systems such as viruses or other pathogens while maintaining full control of shape and structure [16] . Indeed, ligand valencies beyond 32 ( [9] , [18] ) have not been possible before with full control (Indeed, valencies >100 are rare in any glycodendrimeric structure. See the following references André et al. [22] and Camponovo et al. [23] for examples of 128-mer lactoside and 243-mer xyloside display, respectively.) [22] , [23] . We have previously demonstrated that symmetrically multivalent glycan ligands mounted on protein platforms (glycodendriproteins) are useful tools to study carbohydrate–protein interactions and are able to control or modulate a desired response [24] , [25] , [26] , [27] . Other dendrimeric displays on proteins have also been explored subsequently [28] , [29] , [30] . However, to date, this approach has provided only limited carbohydrate valency levels on single protein platforms. We envisaged that a controlled design for a highly polyvalent protein display of sugars might be achieved through a novel strategy of ‘nested polyvalency’ (polyvalent display of polyvalency) ( Fig. 1a ). 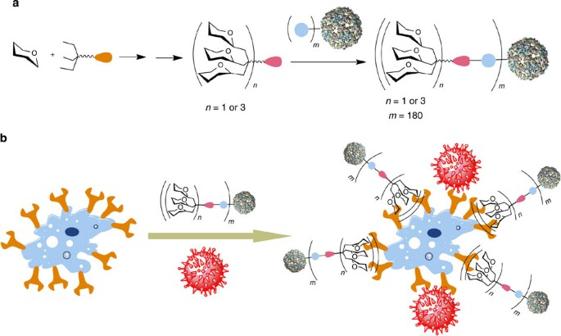Figure 1: Schematic representation of the nested polyvalency strategy. (a) Nested symmetrical assembly of virus-like glycodendrinanoparticles using a tag-and-modify strategy. Glycodendrons are created through iterative multivalent assembly and then attached to multiple tags, each in a monomer protein. (b) Ebola (shown in red) infection model and its competitive inhibition with virus-like glycodendrinanoparticles. Figure 1: Schematic representation of the nested polyvalency strategy. ( a ) Nested symmetrical assembly of virus-like glycodendrinanoparticles using a tag-and-modify strategy. Glycodendrons are created through iterative multivalent assembly and then attached to multiple tags, each in a monomer protein. ( b ) Ebola (shown in red) infection model and its competitive inhibition with virus-like glycodendrinanoparticles. Full size image We describe here the realization of this approach through the multivalent assembly of protein monomers themselves carrying polyvalent glycan display motifs (glycodendrons). The resulting glycodendriprotein homomultimers display many glycans in a precise manner. Consistent with associated guiding physical principles [31] , [32] , [33] , these constructs therefore display symmetry and pseudosymmetry at both the level of protein assembly and glycodendron. These synthetic glycoprotein assemblies display the highest known number of glycans ( n =1,620) yet presented in a homogeneous manner. We have applied this idea ( Fig. 1 ) here to the inhibitory immunomodulation of a DC-SIGN-pathogen glycoprotein interaction ( Fig. 1b ). Construction of glyco-dendri-protein-nano-particles We reasoned that assembly of an entity with similar dimensions (in the form of a self-assembled protein sphere-like icosahedron Qβ [34] , ~28 nm in diameter) might mimic the display in target pathogens (Ebola pseudotyped virus particles have ~90 nm in diameter). Using a tag-and-modify [27] strategy, we chose to selectively introduce a non-natural amino acid (tag) on the protein that could be used for the attachment (modify) of the selected glycodendrons appropriately functionalized at the focal position. As a stringent test of this approach we chose to mimic the highly glycosylated pathogen envelopes of Ebola virus. We selected a monomer Qβ [34] , [35] protein as carrier, which assembles into a 180-copy multimer. Qβ multimer has been used by us and others to display glycans for other purposes but in these prior experiments only partial levels of nonspecific modification were achieved (see Supplementary Discussion ). The result of these prior incomplete reactions was a formation of mixtures and not the desired homogeneous and (pseudo)symmetrical display required for this study [36] , [37] . This proteic platform provided the necessary viral mimic scaffold (core diameter, ~28 nm) [34] to construct the desired multivalent systems. The designed glycodendrons were prepared in a straightforward manner by the Cu(I)-catalysed modification [38] , [39] of the Huisgen cycloaddition as depicted in Fig. 2 . α- D -Mannose was chosen to be introduced onto the dendritic scaffolds as a relevant ligand that is recognized by DC-SIGN [5] . Synthesis of glycodendron 4 was accomplished using a modular strategy that advantageously avoided the need for carbohydrate protection. First, unprotected azidoethyl mannoside 3 (see Supplementary Methods ) [8] was coupled to the trialkynyl pentaerythritol core 2 using CuSO 4 and sodium ascorbate in a 1:1 mixture of water:THF (tetrahydrofuran) at room temperature (RT) [40] . The focal azido group required for subsequent site-specific conjugation to the protein tag, was introduced by reaction with sodium azide to give 5 . The designed modular strategy also allowed use of 5 in the construction of higher generation glycodendron 8 . Thus, coupling of 5 with the trialkynyl core 6 gave 7 ( Fig. 2 ), which was similarly converted to an azide 8 for protein modification. 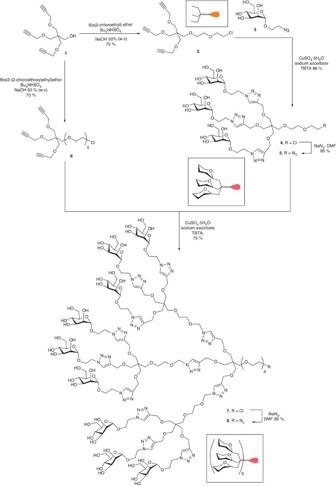Figure 2: Creation of polyvalent mannose-terminated glycodendrons. Synthesis of the glycondendron reagents5and8used in the assembly of virus-like glycodendri-nano-particles (seeFig. 3). TBTA, tribenzyl(tris)triazoylamine; DMF,N,N-dimethylformamide. Figure 2: Creation of polyvalent mannose-terminated glycodendrons. Synthesis of the glycondendron reagents 5 and 8 used in the assembly of virus-like glycodendri-nano-particles (see Fig. 3 ). TBTA, tribenzyl(tris)triazoylamine; DMF, N , N -dimethylformamide. Full size image Unnatural alkyne-containing amino acid L -homopropargylglycine (Hpg) was site-specifically introduced into the protein that would make up the proteic scaffold (Qβ) to serve as an alkyne ‘tag’ through the expression of corresponding gene sequences in an auxotrophic strain of E. coli (B834(DE3)) [41] . Gene sequences were designed to create a protein displaying alkyne at a site on the outer surface of the eventual icosahedral platform (Hpg16) for which the position could simply be controlled by the ‘Met’ triplet codon ATG. Replacement of wildtype methionine (Met) residues, with near-isosteric amino acid isoleucine allows reassignment of the codons in the gene sequence to allow incorporation instead of Hpg as a ‘tag’ (see Supplementary Methods for full details). The resulting Qβ-(Hpg16) 180 was characterized, including by mass spectrometry and dynamic light scattering ( Fig. 3 and see Supplementary Methods and Supplementary Fig. S1 ), demonstrating the introduction of the Hpg amino acid into the sequence. On the basis of previous results [42] , [43] , Qβ-(Hpg16) 180 was modified using a reaction mixture of Cu(I)Br complexed by tris[(1-ethylacetate-1 H -1,2,3-triazol-4-yl)methyl]amine in acetonitrile ( Fig. 3a ). It should be noted that the presence of Hpg on the protein results in slower Huisgen cycloaddition reaction rates in comparison with those obtained when azide in the form of azidohomoalanine (Aha) is present in the protein [42] , [43] . Optimization of the reaction conditions by varying catalyst loading and stepwise addition, afforded the desired glycodendron-bearing virus-like particles. Thus, reaction of Qβ-(Hpg16) 180 with trivalent glycodendron 5 afforded Qβ-(Man 3 ) 180 bearing 540 terminal mannosyl residues and reaction with second-generation nonavalent glycodendron 8 gave Qβ -(Man 9 ) 180 . Both reactions proceeded with >95% conversion; consistent with greater bulk a longer reaction time (up to 7.5 h) was required for reaction of 8 to form 1,620-mer Qβ- (Man 9 ) 180 . Increasing particle diameter was observed, Qβ (27.6 nm)→Qβ-(Man 3 ) 180 (29.8)→Qβ-(Man 9 ) 180 (32.0), consistent with the controlled introduction of ‘shells’ of glycosylation ~1.1 nm thick ( Fig. 3b and see Supplementary Table S1 for rough estimate of dendron length) for each dendron generation. To the best of our knowledge, this is the first synthesis reported of such highly functionalized monodisperse glycodendriproteins (bearing up to 1,620 terminal sugar moieties) using a convergent approach. 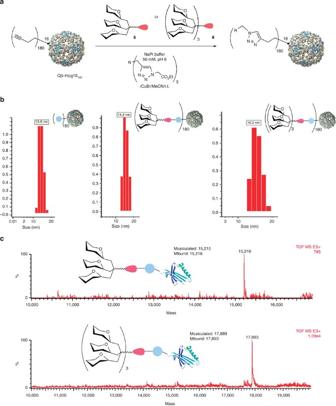Figure 3: Controlled assembly and characterization of virus-like glycodendri-nano-particles. (a) A tag-and-modify strategy allowed the generation of the second nested layer of multivalency from Qβ-(Hpg16)180using glycondendron reagents5and8. R=corresponding glycodendron. (b) Dynamic light scattering histograms showing the hydrodynamic radius of Qβ (radius 13.8 nm), Qβ-(Man3)180(radius 14.9) and Qβ-(Man9)180(radius 16.0). (c) Mass spectrometric analysis of monomer proteins of the particles. Pi, phosphate. Figure 3: Controlled assembly and characterization of virus-like glycodendri-nano-particles. ( a ) A tag-and-modify strategy allowed the generation of the second nested layer of multivalency from Qβ-(Hpg16) 180 using glycondendron reagents 5 and 8 . R=corresponding glycodendron. ( b ) Dynamic light scattering histograms showing the hydrodynamic radius of Qβ (radius 13.8 nm), Qβ-(Man 3 ) 180 (radius 14.9) and Qβ-(Man 9 ) 180 (radius 16.0). ( c ) Mass spectrometric analysis of monomer proteins of the particles. P i , phosphate. Full size image Inhibition of DC-SIGN in vitro and on T lymphocytes The inhibitory function of these glycodendriprotein particles was tested in several ways. Competition ELISA assay (See Supplementary Methods and Supplementary Figs S2 and S3 ) revealed that Qβ-(Man 3 ) 180 could completely inhibit the binding of DC-SIGN (as an Fc chimera) to a synthetically mannosylated glycoprotein (albumin bearing Manα1–3(Manα1–6)Man) with an estimated IC 50 ~35–40 nM. A complete lack of inhibition by control, non-glycosylated Qβ confirmed dependence of this promisingly potent inhibition upon glycan. Next, an Ebola viral infection model [44] , was explored using mammalian T-lymphocyte (Jurkat) cells displaying DC-SIGN. Recombinant viruses were produced in HEK 293 T cells; the viral construction was pseudotyped with Ebola virus envelope GP (EboGP) or the vesicular stomatitis virus envelope glycoprotein (VSV-G) and expressed luciferase as a reporter of the infection [45] . The inhibition of DC-SIGN-dependent infection of T-lymphocyte Jurkat cells (examined in at least three independent experiments) demonstrated that unglycosylated Qβ reduced infection minimally ( Fig. 4a ). In contrast, Qβ-(Man 3 ) 180 and Qβ-(Man 9 ) 180 showed strong dose-dependent inhibition of the infection process ( Fig. 4a–c ). Indeed, Qβ-(Man 9 ) 180 presented a notable antiviral activity, inhibiting infection by ~80% at 5 nM; estimated IC 50 s=9.62 nM for β-(Man 3 ) 180 and=910 pM for Qβ-(Man 9 ) 180 . 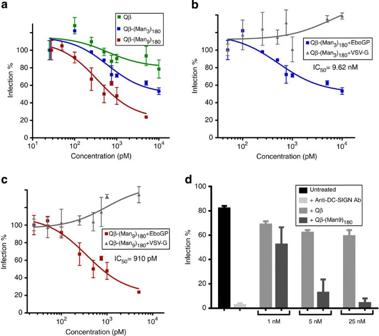Figure 4: Inhibition of viral infection of mammalian cells. (a) Comparison of infection rates of T-lymphocyte (Jurkat) cells displaying DC-SIGN by EboGP pseudovirus in the presence of Qβ, Qβ-(Man3)180, Qβ-(Man9)180; (b) Inhibition by Qβ-(Man3)180of EBOV-GP (EboG) pseudovirus and vesicular stomatitis psuedovirus (VSV-G) in the infection (% infection)of T-lymphocyte (Jurkat) cells displaying DC-SIGN; (c) as for (b) using Qβ-(Man9)180. Values correspond to means of three experiments with s.e.m. shown; the IC50s were estimated using Graphpad Prism v4.0 at 95% with a 95% confidence interval (4.43–20.9 nM for Qβ-(Man3)180and 651 pM–1.3 nM for Qβ-(Man9)180) and settings for normalized dose-response curves. See theSupplementary Fig. S5for duplicated inhibition assays. (d) Inhibition of infection incisof human DCs by EBOV-GP (EboG) using Qβ-(Man9)180. Anti-DC-SIGN Ab is an antibody that blocks DC-SIGN. Immature DCs were generated from isolated human PBMCs. Blockade with anti-DC-sign antibody was used as a positive control. Figure 4: Inhibition of viral infection of mammalian cells. ( a ) Comparison of infection rates of T-lymphocyte (Jurkat) cells displaying DC-SIGN by EboGP pseudovirus in the presence of Qβ, Qβ-(Man 3 ) 180 , Qβ-(Man 9 ) 180 ; ( b ) Inhibition by Qβ-(Man 3 ) 180 of EBOV-GP (EboG) pseudovirus and vesicular stomatitis psuedovirus (VSV-G) in the infection (% infection)of T-lymphocyte (Jurkat) cells displaying DC-SIGN; ( c ) as for ( b ) using Qβ-(Man 9 ) 180 . Values correspond to means of three experiments with s.e.m. shown; the IC 50 s were estimated using Graphpad Prism v4.0 at 95% with a 95% confidence interval (4.43–20.9 nM for Qβ-(Man 3 ) 180 and 651 pM–1.3 nM for Qβ-(Man 9 ) 180 ) and settings for normalized dose-response curves. See the Supplementary Fig. S5 for duplicated inhibition assays. ( d ) Inhibition of infection in cis of human DCs by EBOV-GP (EboG) using Qβ-(Man 9 ) 180 . Anti-DC-SIGN Ab is an antibody that blocks DC-SIGN. Immature DCs were generated from isolated human PBMCs. Blockade with anti-DC-sign antibody was used as a positive control. Full size image VSV-G is able to infect T-lymphocyte Jurkat cells independently of DC-SIGN [44] and provided a positive control in infection experiments; consistent with the proposed model of inhibition ( Fig. 1 ) this glycan-independent pathway for VSV-G was completely uninhibited ( Fig. 4b ). In this model, the Ebola infection process is absolutely dependent on the presence of DC-SIGN on the cell surface. Jurkat cells not expressing DC-SIGN were used as a negative control in the infection studies and showed no infection by Ebola pseudovirus (See Supplementary Fig. S4 ). The ratio of infection in cis between Jurkat DC-SIGN+ and Jurkat cells was ~2,600 for Ebola virus infection and 0.96 for VSV infection. Blocking of DC infection by pseudotyped Ebola Having shown such potent inhibition of infection of a stable cell line that displays DC-SIGN, we next evaluated inhibition in the perhaps more relevant and more demanding context of inhibition of primary cells. DCs are a primary target of Ebola infection; these display multiple C-type lectins that could provide a different or modulated route for infection with potentially higher affinty for virus. Accordingly, DCs were generated from isolated human peripheral blood mononuclear cells (PBMCs) and tested. We were pleased to find that as for the stable Jurkat cell line presenting DC-SIGN alone, Qβ-(Man 9 ) 180 displayed potent activity ( Fig. 4d ), inhibiting infection by >80% at 5 nM and >95% at 25 nM (estimated IC 50 ~2 nM for Qβ-(Man 9 ) 180 ). Excitingly, these data indicate that the mode of inhibition of these synthetic glycodendrinanoparticles translates into cellular contexts relevant to human infection and are consistent with the mode of action suggested in Fig. 1 . Although the evaluation of the number of monomer units interacting during these inhibitory processes is complicated by quasi-equivalence [32] , the data obtained indicate that these systems afford a clear polyvalency effect (β) [46] when compared with the monomer methyl α- D -mannopyranoside) (see Supplementary Table S2 ). The inhibitory properties of each mannoside monomer unit can therefore be considered [46] to be ~250-fold and ~860-fold (as judged by β/N, see Supplementary Table S2 ) more potent when displayed in Qβ(Man 3 ) 180 and Qβ-(Man 9 ) 180 , respectively, than when displayed alone. The efficiency of this system therefore relies upon a vital combination of not only a high number of displayed ligands but also display size and geometry. To date, no homogeneous polyvalent systems have been described that can generate such a large surface area (solvent-accessible surface area ~725,000 Å 2 [47] ) as the systems we have described here. The system we describe here is based on an icosahedral scaffold ( T =3, triakis iscosahedral) that generates several underlying quasi-symmetry elements including those that relate the displayed glycodendrons in a two-fold, three-fold and six-fold manner (see Supplementary Movie 1 ). It is tempting to speculate that this, in turn, allows the simultaneous display of many distinct putative global glycan clusters where the glycan ‘tips’ are also quasi-equivalent (for example, 6-fold-related faces displaying a resultant 54-mer in Qβ-(Man 9 ) 180 or a 3-fold-related 9-mer in Qβ-(Man 3 ) 180 , see Supplementary Movie 1 ). In this way, the nested glycan polyvalency that we have developed here may allow many subtly varying polyvalent combinations to be displayed, each of which (or even a combination of which) might give rise to optimal biological function (here inhibition of Ebola binding). These constructs are therefore not ‘balls of sugar’ but homogenous constructs that array varying faces with different polyvalent glycan arrangements. Thus, their most relevant structural features may well not be simply their average glycan-to-glycan distance (as estimated, say, from Cα-to-Cα residue distances of ~28–40 Å for 2-fold up to 6-fold quasi-symmetry) but instead the specific topology of glycan display and how that relates to both the inter-domain distances in the DC-SIGN tetramer [48] as well as its organization on cell surfaces. [49] Moreover, initial inspection of other viral surfaces suggests that such topologies might effectively out-compete not only Ebola but also other human pathogens. The striking β values that we have discovered here may well arise from such specific ‘optimal’ faces (see Supplementary Movie 1 for illustrative examples of these quasi-symmetrical faces). Indeed, although direct comparison with non-viral systems is not possible, non-viral particles displaying multiple mannosyl residues in a less ordered manner are notably less potent and show much lower multivalency effects (β≤20, see Supplementary Table S2 ). In summary, a novel nested polyvalency approach combined with tag-and-modify site-selective protein synthesis has allowed the creation of homogeneous protein platforms bearing glycodendrons. These well-defined polyvalent glycoprotein assemblies present on their surface up to 1,620 copies of glycan, a remarkably high valency never obtained before using a fully controlled strategy. These glycodendriprotein particles show exciting antiviral activity, preventing mammalian cell infection by Ebola pseudotyped virus through competitive blockade of the DC-SIGN receptor in the nanomolar to picomolar range. These results clearly indicate the efficiency of these systems to interact with this pattern recognition receptor and to compete with pathogens during their entry into target cells. Their in vivo activity remains to be tested and it is possible that such constructs, if used in this context, could elicit humoral responses that might potentially neutralize some of the interactions studied here. The high activity and fascinating (quasi)symmetric, high surface area morphology of these new glycoconjugates provides promising candidates for the development of both new antiviral agents as well as probes of larger-scale biological events. Synthesis of glycodendrons Glycodendron 4 : 2-Azidoethyl α- D -mannopyranoside (306 mg, 1.2 mmol), 2-(2-chloroethoxy)ethoxymethyl trikis(2-propynyloxymethyl)methane (128 mg. 0.37 mmol), CuSO 4 ·5H 2 O (9 mg, 0.04 mmol), tribenzyl(tris)triazoylamine (39 mg, 0.07 mmol) and sodium ascorbate (29 mg, 0.15 mmol) were dissolved in 2 ml of THF/H 2 O (1:1). After consumption of the starting material (3 h), the solvent was evaporated and the crude was purified by size-exclusion chromatography (Sephadex LH-20 MeOH 100%), furnishing the glycondendron 4 as a white foam (347 mg, 86%). Glycodendron 5 : Glycodendron 4 (80 mg, 0.07 mmol) and sodium azide (47 mg, 0.7 mmol) were dissolved in N , N -dimethylformamide (2 ml). The mixture was stirred at 60 °C for 4 days. After consumption of the starting material, the solvent was concentrated and the crude was purified by size-exclusion chromatography (Sephadex G-25 H 2 O/MeOH 9:1), furnishing glycondendron 5 (76 mg, 95%) as a white foam. Glycodendron 7 : Glycodendron 5 (30 mg, 0.03 mmol), [2-[2-(2-chloroethoxy)ethoxy]ethoxy]ethoxymethyl tris(2-propynyloxymethyl)methane (3.6 mg, 0.008 mmol), CuSO 4 ·5H 2 O (0.5 mg, 0.002 mmol), tribenzyl(tris)triazoylamine (1.7 mg, 0.003 mmol) and sodium ascorbate (1.3 mg, 0.006 mmol) were dissolved in THF/H 2 O (1:1, 1 ml). After consumption of the starting material, the solvent was evaporated and the crude was purified by size-exclusion chromatography (Sephadex LH-20 MeOH 100%), furnishing glycondendron 7 (22 mg, 75%) as a white foam. Glycodendron 8 : Glycodendron 7 (25 mg, 0.007 mmol) and sodium azide (4 mg, 0.07 mmol) were dissolved in N , N -dimethylformamide (1 ml). The mixture was stirred at 60 °C for 4 days. After that, the solvent was concentrated and the crude was purified by size-exclusion chromatography (Sephadex G-25 H 2 O/MeOH 9:1), furnishing glycondendron 8 (20 mg, 80%) as a white foam. Synthesis of virus-like glycodendrinanoparticles Glycoprotein Qβ-(Man 3 ) 180 : Glycodendron 5 (2.84 mg, 0.002 mmol) was dissolved in sodium phosphate buffer (50 mM, pH=8, 200 μl). Protein solution (180 μg, 100 μl) was added to the above solution and mixed thoroughly. A freshly prepared solution of copper (I) bromide (99.999%) in acetonitrile (32.6 μl of 10 mg ml −1 ) was premixed with an acetonitrile solution of tris[(1-ethylacetate-1 H -1,2,3- triazol-4-yl)methyl] amine (12.6 μl of 100 mg ml −1 ). The preformed Cu-complex solution (25 μl) was added to the mixture and the reaction was agitated on a rotator for at RT. After 4 h, 150 μl of buffer and 50 μl of fresh Cu-complex solution were added to the mixture again and the reaction was agitated for a further 1.5 h. The resulting mixture was purified in PD-MiniTrap (G-25) twice and concentrated on a vivaspin membrane concentrator (30 KDa molecular weight cut off) to 400 μl. To a virus-like particle aliquot (20 μl) was added 1 μl of TCEP (1 M) to allow the protein to denature before analysis by liquid chromatography–mass spectrometry. Electrospray Ionization Mass Spectrometry (TOF ES+) ( m/z ): calc. 15,215; found 15,216. Glycoprotein Qβ-(Man 9 ) 180 : Glycodendron 8 (4.8 mg, 0.001 mmol) was dissolved in sodium phosphate buffer (50 mM, pH=8, 50 μl). Protein solution (90 μg, 50 μl) was added to the above solution and mixed thoroughly. A freshly prepared solution of copper (I) bromide (99.999%) in acetonitrile (32.6 μl of 10 mg ml −1 ) was premixed with an acetonitrile solution tris[(1-ethylacetate-1 H -1,2,3- triazol-4-yl)methyl] amine, (12.6 μl of 100 mg ml −1 ). The preformed Cu-complex solution (25 μl) was added to the mixture and the reaction was agitated on a rotator at RT. After 3 and 6 h, 50 μl of buffer and 12.5 μl of fresh Cu-complex solution were added to the mixture again (each time) and the reaction was agitated for further 1.5 h. The resulting mixture was purified in PD-MiniTrap (G-25) twice and concentrated on a vivaspin membrane concentrator (30 KDa molecular weight cut off) to 400 μl. To a virus-like particle aliquot (20 μl) was added 1 μl of TCEP (1M) to allow the protein to denature before analysis by liquid chromatography–mass spectrometry. ESI-MS (TOF ES+) ( m/z ): calc. 17,889; found 17,893. Production of recombinant viruses Recombinant viruses were produced in 293T cells. The viral construction was pseudotyped with EboGP or VSV-G and expressed luciferase as a reporter of the infection [45] . One day (18–24 h) before transfection, 6 × 10 6 293T were seeded onto 10 cm plates. Cells were cultured in DMEM medium supplemented with 10% heat-inactivated FBS, 25 mg gentamycin, 2 mM L -glutamine. A few minutes before transfection, the medium on transfection plates was changed to 9 ml DMEM and chloroquine was added to 25 μM final concentration. Transfection reaction with all reagents at RT was prepared in 15 ml tubes: 183 μl of 2M CaCl 2, 450 ng of Ebola virus envelope, 21 μg of pNL4-3 luc [50] , 1,300 μl of water. Next, 1.5 ml of 2xHBS (hepes buffer saline) pH 7.0 was added quickly to the tubes and bubbled for 30 s. HBS/DNA solution was gently dropped onto medium. After 8 h of incubation at 37 °C with 5% CO 2 , medium on transfection plates was changed to 10 ml DMEM and once again 1 day after transfection to 7 ml DMEM. Transfection supernatants were collected after 48 h, centrifuged at 1,200 rpm for 10 min at RT to remove cell debris, and stored frozen at −80 °C (ref. 51 ). Infection of Jurkat cells displaying DC-SIGN in cis Infection was performed on Jurkat cells (T-lymphocyte cell line) expressing receptor DC-SIGN on their surface. One day before infection, 5 × 10 4 of Jurkat DC-SIGN cells were plated into each well of 96-well plate. Cells were incubated at RT for 20 min with the carbohydrate-based compounds and then challenged with 5000 Tissue Culture Infective Dose of recombinant viruses. After 48 h of incubation cells were washed twice with PBS and lysed for luciferase assay. The range of concentrations tested for compounds Qβ and Qβ-(Man 3 ) 180 was 100 pM–50 nM and for compound Qβ-(Man 9 ) 180 was 50 pM–50 nM. As a control, an experiment of infection with VSV-G pseudoviruses was performed under the same conditions. Infection with VSV-G is independent of the presence of DC-SIGN receptor. Generation of monocyte-derived DCs (DCs) PBMCs were isolated from buffy coats from healthy human donors (Hospital 12 de Octubre, Madrid, Spain) by Ficoll-Paque (Pharmacia, Uppsala, Sweden) density-gradient centrifugation. Following the centrifugation of 40 ml of whole blood samples on Ficoll-Paque at 2,000 rpm for 30 min, the cells from interface were collected and washed five times with PBS at 1,500 rpm for 5 min at RT. PBMCs were then resuspended in RPMI medium supplemented with 10% heat-inactivated FBS, 25 mg gentamycin, 2 mM L -glutamine at concentration 2 × 10 6 cells per ml and placed onto 24-well plate for 1 h at 37 °C with 5% CO 2 . The adherent monolayer of monocytes were then washed twice with PBS and resuspended in RPMI medium supplemented with cytokines granulocyte–macrophage colony-stimulating factor (200 ng ml −1 ) and IL-4 (10 ng ml −1 ). For the differentiation of immature monocyte-derived DCs, cells were incubated at 37 °C with 5% CO 2 for 7 days and subsequently activated with cytokines on day 2 and 5 (refs 44 , 52 , 53 ). Infection of immature monocyte-derived DCs in cis Immature monocyte-derived DCs were incubated at RT for 20 min with the carbohydrate-based compounds and then challenged with 5000 TCID of EBOV-GP recombinant pseudoviruses. After 48 h of incubation cells were washed twice with PBS and lysed for luciferase assay. The range of concentrations tested for Qβ-(Man 9 ) 180 was 1, 5 and 25 nM. As a control, experiment of inhibition of infection of EBOV-GP was performed in the presence of antibody anti-DC-SIGN and mannan at concentration of 25 μg ml −1 . Statistical methods Dynamic light scattering : Dynamic light scattering values represent the average of 10 independent measurements, where 10 individual acquisitions were taken per measurement the results analysed using OmniSIZE software. Infection assays : Statistical analysis was performed using GraphPad Prism v6.0. Infection of mammalian Jurkat cells displaying DC-SIGN by EboV-GP pseudotyped viruses : The values of percentage of infection presented on the graph correspond to the mean of six independent experiments with error bars corresponding to the s.e.m. The IC 50 values were estimated using GraphPad Prism v6.0 with a 95% confidence interval and settings to normalize dose-response curves. Infection of primary monocyte-derived DC by EboV-GP pseudotyped viruses : The values of percentage of infection correspond to the mean of two independent experiments (error bars describe the range between the two values obtained). How to cite this article: Ribeiro-Viana, R. et al. Virus-like glycodendrinanoparticles displaying quasi-equivalent nested polyvalency upon glycoprotein platforms potently block viral infection. Nat. Commun. 3:1303 doi: 10.1038/ncomms2302 (2012).